Monolithic nonlinear pulse compressor on a silicon chip Projected demands in information bandwidth have resulted in a paradigm shift from electrical to optical interconnects. Switches, modulators and wavelength converters have all been demonstrated on complementary metal-oxide semiconductor compatible platforms, and are important for all optical signal and information processing. Similarly, pulse compression is crucial for creating short pulses necessary for key applications in high-capacity communications, imaging and spectroscopy. In this study, we report the first demonstration of a chip-scale, nanophotonic pulse compressor on silicon, operating by nonlinear spectral broadening from self-phase modulation in a nanowire waveguide, followed by temporal compression with an integrated dispersive element. Using a low input peak power of 10 W, we achieve compression factors as high as 7 for 7 ps pulses. This compact and efficient device will enable ultrashort pulse sources to be integrated with systems level photonic circuits necessary for future optoelectronic networks. In the rapidly evolving fields of computing and telecommunications, higher data rates are needed to keep pace with the demands on data bandwidth. Replacing electrical interconnects with optical interconnects [1] , [2] , [3] , [4] , [5] , [6] implemented on complementary metal-oxide semiconductor (CMOS)-compatible photonic integrated circuits provides one of the most promising and cost-effective ways to meet these demands. Extensive research efforts have been focused on all optical functionalities for wavelength division multiplexing, including on-chip optical parametric oscillators [5] and wavelength conversion [6] . Similar to wavelength division multiplexing, optical time division multiplexing (OTDM) provides an efficient means to tremendously enhance the capacity of a transmission medium by interleaving several low-rate data streams in time to produce a single data stream at higher rates which can exceed 1 Tbit s −1 (refs 7 , 8 , 9 ). Crucial to the implementation of ultrafast OTDM are short pulses, the generation of which is not trivial. Consequently, temporal compression [10] , [11] is necessary to obtain short pulses from a longer pulse source. These short pulses derived from temporal compression are also essential for diverse applications, including optical coherence tomography [12] and time-resolved spectroscopy [13] . Such compression has been demonstrated in fibre-based systems, including silica [11] , [14] , microstructure [15] and chalcogenide fibres [16] . However, these systems lack compactness and are contrary to the general theme of CMOS-compatible photonic integrated circuits. Furthermore, fibre-based compression systems generally require operation at higher powers to offset the weak third order nonlinearity in the host material. Although chip scale pulse compression based on high-order solitons has recently been demonstrated [17] , [18] , [19] , the requisite high-compression factors (defined as the ratio of the output and input pulse full-width at half-maximum (FWHM)) required for practical applications including ultrafast OTDM has yet to be realized on a CMOS-compatible integrated platform. Fundamental to pulse compression is the acquisition of nonlinear phase through self-phase modulation [20] . The third order susceptibility of the host material results in an intensity-dependent phase shift, which leads to the creation of new optical frequencies. When appropriately combined with optical dispersion, pulse compression results. This dispersion may be distributed over the length of the nonlinear medium, leading to solitonic compression, or may be localized at the output of the nonlinear medium using a highly dispersive element. We recently reported the theory and operation of such a dispersive element in silicon [21] , [22] , thus opening up vast prospects for all-optical on-chip functionalities for which dispersion is a key requirement. Such an element has been absent in the on-chip nanophotonics toolkit, and to date, most integrated optics applications requiring dispersive elements required heterogeneous integration with fibre-based components, resulting in less compact systems. In this study, we demonstrate for the first time, a chip scale, compact, monolithically integrated nonlinear pulse compressor operating via self-phase modulation in a silicon nanowire waveguide, followed by re-phasing with an integrated dispersive element. We report optimal compression factors as high as 7 at a low input peak power of 10 W. The requisite large acquired nonlinear phase for high compression factors is obtained at low input peak powers, owing to the large third order Kerr nonlinearity in silicon, high modal confinement in the carefully designed nanowire waveguide and, consequently, large nonlinear parameter, γ [20] , [23] , [24] , [25] , [26] . 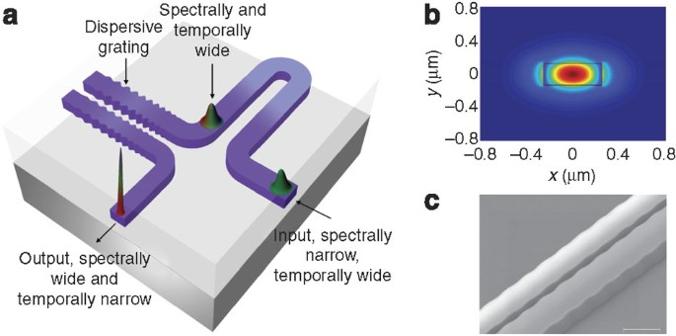Figure 1: Schematic of the nonlinear pulse compressor. (a) Pulses at the input are spectrally broadened because of self-phase modulation via the Kerr nonlinearity in the highly confined silicon nanowire waveguide. The pulses are then compressed by the dispersive grating leading to spectrally wide and temporally narrow output pulses. (b) Calculated quasi-TE mode profile for silicon nanowire waveguide used for self-phase modulation. (c) Scanning electron micrograph of dispersive grating before deposition of SiO2overcladding. The scale bar represents a length of 500 nm. Design and modelling of nonlinear pulse compressor The schematic of our nonlinear pulse compressor is shown in Figure 1a . Pulses at the input propagate through a 6-mm silicon nanowire waveguide (250 nm by 500 nm), which is cladded with SiO 2 and undergoes self-phase modulation. Figure 1b shows the cross-section and the calculated quasi-TE (transverse electric) mode profile for the nanowire waveguide. The output of the nanowire waveguide enters a dispersive grating ( Fig. 1c ), which will provide the quadratic phase necessary to compensate for the frequency chirp acquired in the nanowire waveguide and in so forth, bring about pulse compression. As illustrated in Figure 1a , the self-phase modulation process will generate red-shifted and blue-shifted frequencies at the leading and trailing edge of the pulse, respectively [20] . The anomalously dispersive grating is necessary to delay the red-shifted component and advance the blue-shifted component to approach a transform-limited pulse. The dispersive grating consists of two coupled, sinusoidally corrugated waveguide gratings [21] , [22] with different average widths for cross coupling of the forward propagating wave at the input waveguide and the backward propagating wave at the output waveguide to occur. A positive, linearly chirped period is applied to generate the required anomalous dispersion across the transmission bandwidth. The large Kerr nonlinearity and small effective area (0.15 μm 2 ) in our highly confined silicon nanowire waveguide enables significant self-phase modulation-induced nonlinear phase shift at low input powers and using short lengths. The calculated group velocity dispersion of the nanowire waveguide is 1070 ps nm −1 km −1 at 1.55 μm, implying dispersion lengths much larger than the waveguide length for pulses on the picosecond scale. Therefore, the pulse dynamics are negligibly affected by the waveguide dispersion. We note that the negligible dispersive effect in the waveguide leads to a slightly lower compressed pulse quality, but to higher compression factors as compared with normally dispersive media with comparable dispersive and nonlinear lengths [11] . Using the split-step Fourier method, the dynamics of the nonlinear pulse compressor using 7 ps FWHM Gaussian pulses as the input are studied by numerically solving the nonlinear Schrödinger equation [20] . Pulse evolution is monitored as a function of input peak power ( Fig. 2a ). For clarity, the input peak power referred to in this manuscript refers to the peak power coupled to the waveguide input, normalized to the fibre-waveguide coupling loss. We use a value of grating dispersion, which is measured in the next section. For a fixed dispersive grating length, optimal compression is obtained when the frequency chirp acquired by a pulse with a specific, optimum peak power is maximally compensated for by the grating dispersion, and we obtain a pulse closest to transform limited. 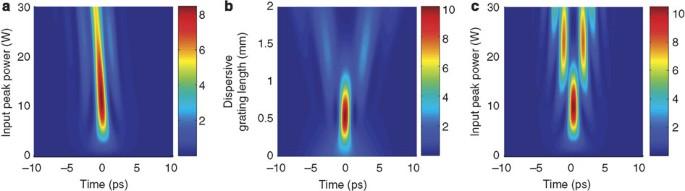Figure 2: Numerical results of the nonlinear pulse compressor using the nonlinear Schrödinger equation. (a) Pulse intensity profile as a function of coupled input peak power for a fixed grating length of 500 μm. The advancement in time and increasing pulse asymmetry is a result of FCA. (b) Pulse intensity profile as a function of grating length for a fixed input peak power of 10 W. A multilobed profile develops as the grating length is increased due to the excess dispersion. (c) Pulse intensity profile as a function of coupled peak power for a fixed grating length of 500 μm in the absence of free carriers. The pulse evolves symmetrically without advancing in time. Pulse splitting is apparent at higher peak powers because of the larger acquisition of nonlinear phase shift as compared with the case in the presence of free carriers. Referring to Figure 2a , pulse duration is observed to decrease initially as low peak powers are increased up to the optimal peak power of ~10 W, resulting in an output pulse FWHM of 1.1 ps. This is accompanied by an increase in peak power of the output pulses. Below the optimal peak power, the pulses have a single lobe and decrease steadily in duration as the power is increased. A decreasing compression factor observed at low powers is mainly because of the reduction in spectral broadening. At low input peak powers, even though the grating dispersion is smaller than that required to match the acquired nonlinear phase, the deviation of the pulse profile from that for optimal compression is small. This is because the sensitivity of the final pulse duration to the dispersion in the grating is lower for smaller input peak powers as a result of the reduced spectral content. Input pulses above the optimum peak power develop a multilobed profile and although the central lobe of the pulse does not broaden much, the presence of pedestals reduce the overall output peak power of the pulse ( Fig. 2a ). For higher peak powers, the amount of grating dispersion required to bring all frequencies in phase is reduced, and the excess dispersion from the fixed grating length is the cause of the multilobed profile. This effect is also evident in Figure 2b , where the output pulse is studied as a function of the dispersive grating length at a fixed input peak power of 10 W. The pulse broadens and develops pedestals as the grating dispersion used for compression is increased beyond its optimum value. Figure 1: Schematic of the nonlinear pulse compressor. ( a ) Pulses at the input are spectrally broadened because of self-phase modulation via the Kerr nonlinearity in the highly confined silicon nanowire waveguide. The pulses are then compressed by the dispersive grating leading to spectrally wide and temporally narrow output pulses. ( b ) Calculated quasi-TE mode profile for silicon nanowire waveguide used for self-phase modulation. ( c ) Scanning electron micrograph of dispersive grating before deposition of SiO 2 overcladding. The scale bar represents a length of 500 nm. Full size image Figure 2: Numerical results of the nonlinear pulse compressor using the nonlinear Schrödinger equation. ( a ) Pulse intensity profile as a function of coupled input peak power for a fixed grating length of 500 μm. The advancement in time and increasing pulse asymmetry is a result of FCA. ( b ) Pulse intensity profile as a function of grating length for a fixed input peak power of 10 W. A multilobed profile develops as the grating length is increased due to the excess dispersion. ( c ) Pulse intensity profile as a function of coupled peak power for a fixed grating length of 500 μm in the absence of free carriers. The pulse evolves symmetrically without advancing in time. Pulse splitting is apparent at higher peak powers because of the larger acquisition of nonlinear phase shift as compared with the case in the presence of free carriers. Full size image The semiconductor nature of silicon implies a small optical band gap, leading to possible nonlinear losses in the form of two-photon absorption (TPA) and free-carrier absorption (FCA). Because of TPA- and FCA-related losses, an input pulse with high peak power experiences a rapid reduction in its amplitude as it propagates into the silicon nanowire waveguide [23] , [27] , [28] . As the extent of spectral broadening from self-phase modulation scales with the peak power of the pulse, the reduction in pulse amplitude inside the nanowire waveguide limits the final pulse bandwidth and hence the compression factor. In addition, the free carriers generated by the leading edge of the pulse can lead to attenuation of the trailing edge, and concomitant reduction in pulse duration and increase in pulse asymmetry [29] . Consequently, asymmetry of the pulse and temporal advancement of the pulse envelope is observed in Figure 2a to become more significant as the input peak power is increased. For efficient compression, low powers are ideal such that reduction in pulse amplitude and temporal truncation of the pulses is minimal. To further study the detrimental effects of free carriers, we model the pulse evolution as a function of the input peak power, taking into account TPA but in the absence of free carriers. The result is shown in Figure 2c . As expected, the pulses evolve symmetrically without any temporal advancement in the pulse envelope. With the exception of a small power penalty in the presence of free carriers, pulses in the presence ( Fig. 2a ) and absence ( Fig. 2c ) of free carriers evolve in a similar fashion at low input peak powers. However, the free-carrier effects become increasingly significant at higher peak powers. As the density of free carriers scales with the square of the incident intensity, pulse dynamics become FCA limiting at high powers. At input powers exceeding 12 W in the absence of free carriers, pulses acquire a larger nonlinear phase leading to more severe pedestals compared with the case where free carriers are present. Pulse splitting at higher powers observed in Figure 2c is a result of a larger deviation of the dispersion applied from that required to match the generated frequency chirp. In Figure 2a , pulse profiles at higher powers evolve much more slowly as the spectral broadening plateaus off as a result of FCA-induced attenuation of pulse amplitude. The results imply that at higher powers, larger compression factors are achievable in the absence of free carriers when combined with a dispersive grating optimized to match the larger acquired nonlinear phase. Measurement of dispersive grating To demonstrate pulse compression, we design the dispersive grating to provide both the bandwidth and dispersion required to compensate for the frequency chirp generated by self-phase modulation. Details of the dispersive grating design are described in Methods. To characterize the spectral properties of the dispersive grating, we design an integrated Mach-Zehnder interferometer [30] (MZI) for operation with TE-polarized light. The interferometer consists of a directional coupler to split the input field into two arms, one consisting of a 500-μm-long dispersive grating and a second arm consisting of a silicon nanowire reference waveguide (250 nm by 500 nm) with length, L ref =3 mm, followed by another directional coupler at the output to recombine fields from the two arms. 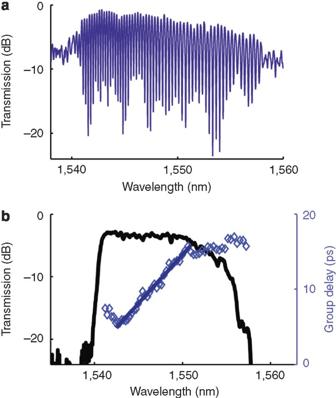Figure 3: Characterization of dispersive grating. (a) Oscillations obtained from the integrated Mach-Zehnder interferometer showing an increase in oscillation period at longer wavelengths. (b) Measured transmission (black) of the nonlinear pulse compressor and group delay (blue) of dispersive grating extracted from Mach-Zehnder interferometer (MZI) oscillations. Using a broadband source, the output spectrum is measured using an optical spectrum analyser (OSA), and the result is shown in Figure 3a . Within the transmission bandwidth of the dispersive grating, oscillations in the output spectrum will result due to constructive and destructive interference [30] . Using the generated oscillations across the transmission bandwidth, the path length difference as a function of wavelength can be extracted. Shorter wavelengths entering the dispersive grating device are transmitted first, and therefore have a larger path length difference with the reference arm. The path length difference, L (λ) = λ 2 /(Δ λ . n g ( λ )), where Δ λ is the oscillation period and n g ( λ ) is the group index of the waveguide. The larger period of oscillation towards the red edge of the transmission band is attributed to the shorter path length difference with the reference arm. Finally, the group delay introduced by the dispersive grating, τ ( λ ) is calculated using τ ( λ ) = ( L ref − L ( λ )). n g ( λ )/ c , where c is the speed of light in vacuum. The extracted group delay is plotted in blue in Figure 3b . Within the 3-dB bandwidth of the dispersive grating, the group delay is very linear. Using the gradient of the group delay within the transmission bandwidth, the total calculated group velocity dispersion, D = d τ ( λ )/d λ = 1.3 ps nm −1 for a grating length of 500 μm, corresponding to 2.6×10 6 ps nm −1 km −1 . In deriving the group delay, we assumed that the grating dispersion dominates. We note that the dispersion in the reference waveguide (1070 ps nm −1 km −1 ) is three orders of magnitude smaller than that in the grating and may therefore be neglected. Figure 3: Characterization of dispersive grating. ( a ) Oscillations obtained from the integrated Mach-Zehnder interferometer showing an increase in oscillation period at longer wavelengths. ( b ) Measured transmission (black) of the nonlinear pulse compressor and group delay (blue) of dispersive grating extracted from Mach-Zehnder interferometer (MZI) oscillations. Full size image Experimental characterization of the nonlinear pulse compressor Our nonlinear pulse compressor consists of a 6-mm-long nanowire waveguide (250 nm by 500 nm) with a measured propagation loss of 6 dB cm −1 , and a 500-μm-long dispersive grating, as designed in the previous section. Using a broadband source adjusted for TE polarization, the linear response of the pulse compressor is measured using an OSA and the result is shown as the black curve in Figure 3b . The 3-dB transmission bandwidth obtained is 11 nm. To generate input pulses for compression, 200 fs pulses centred at 1.55 μm are derived from an optical parametric oscillator pumped by a Ti:Sapphire laser at 830 nm at a repetition rate of 76 MHz. The pulses are filtered using a bandpass filter centred at 1.546 μm with 0.5 nm 3-dB bandwidth to generate 7 ps pulses, followed by amplification using an erbium-doped fibre amplifier (EDFA). The pulses are then adjusted for TE polarization before coupling into the nanowire waveguide, which is terminated with inverse tapers to increase coupling efficiency. A small amount of frequency chirp occurs in the EDFA but is negligible compared with that occurring in the silicon nanowire waveguide. Pulses exiting the compressor are spectrally characterized using an OSA. To measure the temporal profile of the pulses, the device output is amplified using a low-noise EDFA before measurement with an autocorrelator. The temporal and spectral output of the EDFA is observed as a function of amplified power to ensure that no nonlinear effects such as soliton formation occur within the amplifier. To characterize the nonlinear pulse compressor, the spectral output is monitored as the input peak power is varied. 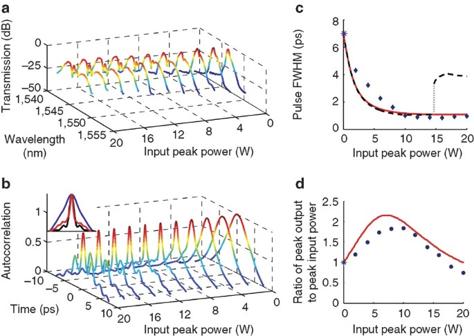Figure 4: Characterization of the nonlinear pulse compressor. (a) Spectral output as a function of input peak power. (b) Autocorrelation traces as a function of input peak power. The inset shows the measured pulse autocorrelation profiles through a 6-mm nanowire waveguide (blue) and through the pulse compressor (red) at an input peak power of 10 W, showing the compression brought about by the combination of nonlinear phase shift and linear dispersion in the grating. The calculated autocorrelation of pulses at the output of the pulse compressor at a peak power of 10 W is displayed as the black line in the inset. (c) Measured (blue diamonds) and calculated (red line) FWHM of the output pulse as a function of input peak power. Black dashed line denotes calculated output pulse FWHM in the absence of free carriers. A Gaussian deconvolution factor of 1.41 is applied to the autocorrelation FWHM to obtain the pulse FWHM. Star denotes FWHM calculated from measured pulse bandwidth assuming a transform limited pulse. (d) Measured (blue circles) and calculated (red line) ratio of output peak power to input peak power, normalized to coupling and propagation losses, as a function of input peak power. Star denotes measured ratio assuming a 7 ps Gaussian pulse (seeMethods). A maximum is observed at an input peak power of 10 W representing the optimal tradeoff between compression factor and nonlinear losses. Self-phase modulation in the silicon nanowire waveguide is evident in Figure 4a, which shows the spectral broadening increasing with the input peak power. The 3-dB bandwidth of the dispersive grating ( Fig. 3b ) is sufficiently large such that minimal truncation of the spectrally broadened pulses occurs, even up to an input peak power of 20 W. The observed spectral broadening is asymmetric, as expected from free-carrier effects. Figure 4b shows the pulse temporal evolution as the input peak power is increased. Because of the limited autocorrelator scanning range of 15 ps, we were unable to accurately measure the autocorrelation of the pulse at the lowest peak input power (~100 mW). However, from the measured output bandwidth of 0.5 nm at the lowest power level, we estimate a minimum pulse FWHM of 7 ps corresponding to a time-bandwidth product of 0.44. On increasing the peak power, a gradual narrowing of the pulse occurs as theoretically expected from the generation of new frequencies from self-phase modulation. An increase in compression is observed up to an input peak power of 10 W, where a pulse FWHM of 1 ps (assuming a Gaussian deconvolution factor of 1.41) is obtained corresponding to a compression factor of 7 (see red curve in Fig. 4b inset). At this input peak power, the nonlinear phase acquired by the pulse is optimally matched to the phase introduced by the dispersive grating leading to optimal compression. A further increase in input peak power is characterized by an increase in the number and level of sidelobe peaks in the pulse. A slightly shorter pulse FWHM of 900 fs is obtained at a peak input power of 12 W representing a compression factor of 7.8. However, the compression at this power level is not optimal as sidelobes adjacent to the main pulse lobe begin to develop. This is consistent with the theory ( Fig. 2a ), as a larger nonlinear phase shift acquired at higher peak powers will require a smaller amount of dispersion to bring the new spectral components in phase. At higher peak powers, the fixed dispersion introduced by the grating is larger than the optimal value for a minimum time-bandwidth product, and a reduction in compressed pulse quality from the excess dispersion occurs. We expect that nonlinear effects arising from interactions with free carriers will give rise to pulses which are increasingly asymmetric at higher input peak powers. It should be noted that the measured pulse profiles are symmetric owing to the nature of autocorrelation measurement. Figure 4: Characterization of the nonlinear pulse compressor. ( a ) Spectral output as a function of input peak power. ( b ) Autocorrelation traces as a function of input peak power. The inset shows the measured pulse autocorrelation profiles through a 6-mm nanowire waveguide (blue) and through the pulse compressor (red) at an input peak power of 10 W, showing the compression brought about by the combination of nonlinear phase shift and linear dispersion in the grating. The calculated autocorrelation of pulses at the output of the pulse compressor at a peak power of 10 W is displayed as the black line in the inset. ( c ) Measured (blue diamonds) and calculated (red line) FWHM of the output pulse as a function of input peak power. Black dashed line denotes calculated output pulse FWHM in the absence of free carriers. A Gaussian deconvolution factor of 1.41 is applied to the autocorrelation FWHM to obtain the pulse FWHM. Star denotes FWHM calculated from measured pulse bandwidth assuming a transform limited pulse. ( d ) Measured (blue circles) and calculated (red line) ratio of output peak power to input peak power, normalized to coupling and propagation losses, as a function of input peak power. Star denotes measured ratio assuming a 7 ps Gaussian pulse (see Methods ). A maximum is observed at an input peak power of 10 W representing the optimal tradeoff between compression factor and nonlinear losses. Full size image The blue curve in the inset of Figure 4b shows the profile of output pulses from a 6-mm reference nanowire waveguide in the absence of the 500-μm grating for a peak input power of 10 W. Plotted in the same figure is the measured (red) and modelled (black) output pulse autocorrelation at an input peak power of 10 W. As expected, the result shows that the presence of the dispersion applied by the grating is necessary for pulse compression. Figure 4c shows the plots of the measured (blue diamonds) and calculated (red line) output pulse FWHM as a function of input peak power. We observe that as the input peak power is increased, the measured compression factor approaches a plateau value of ~7.7. The observed limit is primarily because of a higher than optimal dispersion introduced by the grating, and secondarily because of TPA and FCA effects in limiting the extent of spectral broadening. This secondary effect is also evident in Figure 4c, where the modelled output pulse FWHM in the presence (red line) and absence of free carriers (black dashed line) is shown to evolve in a similar manner at low powers, indicating that free carriers do not have a dominant role. At higher powers, pulse evolution saturates in the presence of free carriers while continuing to evolve in the absence of free carriers, leading to a discontinuity in the output pulse FWHM at ~15 W, when the compressed pulse pedestals exceed the 50% level. These observations are consistent with free carriers limiting the acquisition of nonlinear phase at high powers. The ratio of the output peak power to the input peak power is measured and the result is plotted in Figure 4d (blue circles), together with the calculated values (red line). The ratio is observed to increase first as the input peak power is increased, consistent with the reduction in pulse duration. The measured ratio is further observed to reach a maximum at an input peak power of 10 W where the compression is optimum, before it starts to steadily fall off again from nonlinear losses. In addition, an increasing amount of energy is carried in the compressed pulse sidelobes at higher input powers further contributing to the reduction in output peak power. The highest ratio of peak output to peak input power is obtained at an input of 10 W, representing optimal compression of the input pulses to a pulse FWHM of 1 ps. The nonlinear pulse compressor demonstrated in this study will be useful for generating short pulses for a myriad of applications. However, in the context of optical information processing, consideration must be given to free carriers and the limitations they pose to realizable data rates. The 76 MHz repetition rate used in this study ensures that the free-carrier lifetime is much shorter than the temporal separation of adjacent pulses. Consequently, free-carrier accumulation, which drastically reduces the input peak power, is precluded. At higher data rates, self-phase modulation is compromized [28] and compression cannot occur. To circumvent this problem, methods such as ion implantation [31] or reverse biased P-I-N junctions [32] may be used to greatly reduce free-carrier lifetimes to below 20 ps and in so forth, eliminate free-carrier accumulation at higher data rates. Furthermore, these methods can reduce FCA limitations on nonlinear phase acquisition at higher peak powers. Yin and Agrawal [28] reported that the relation, ν.τ c ≥0.2, (where ν is the laser repetition rate and τ c is the free-carrier lifetime) should be satisfied for self-phase modulation-induced spectral broadening to take place without detriment [28] . Therefore, by adopting the aforementioned methods to reduce free-carrier lifetimes, our nonlinear pulse compressor may efficiently operate at the commonly used rate of 10 Gbit s −1 before multiplexing in 1.28 Tb s −1 OTDM systems [8] , [9] . As the compression factor scales with the nonlinear phase generated through self-phase modulation, our integrated nonlinear pulse compressor may be readily used to generate sub-picosecond pulses by increasing the effective length [20] of the silicon nanowire waveguide. The 6 dB cm −1 propagation losses in our waveguides may be attributed to sidewall roughness as well as stitching errors during electron-beam writing. Given that the waveguide losses may be realistically reduced to 1 dB cm −1 , longer effective lengths may be implemented to achieve greater compression at similar power levels. For a nanowire waveguide ~2.5 cm in length with 1 dB cm −1 loss, a pulse with a low input peak power of 2.5 W will generate similar amounts of spectral broadening and compression as that demonstrated in our paper for optimal compression. In addition, for the same nanowire waveguide length and input peak power, the dispersive grating may be optimized such that the same compression factor may be achieved using shorter input pulses, to obtain even shorter pulses on the femtosecond scale. The method is therefore scaleable such that it may be used to derive ultrashort pulses for a variety of applications. The fully integrated, compact, monolithic CMOS-compatible design makes it particularly useful for optical interconnects and for realizing ultrafast sources necessary to meet future bandwidth demands. Modelling of the nonlinear pulse compressor Using the split-step Fourier method, the dynamics of the nonlinear pulse compressor using 7 ps pulses as functions of both input peak power and dispersive grating length are studied by numerically solving the nonlinear Schrödinger equation [20] , taking into account two photon and free-carrier effects [23] , [27] , [28] . The waveguide dispersion and effective waveguide modal area were obtained using a fully vectorial beam propagation method. The nonlinear refractive index of silicon used to calculate γ from the effective area was varied within the range of reported values [23] , [24] , [25] , [26] , [27] to obtain the best match to measured data. Experimentally measured values for waveguide propagation losses and grating dispersion were used. The estimated dispersion in the output fibres is also incorporated into the model. Design and fabrication of dispersive grating The dispersive grating used in the nonlinear pulse compressor was implemented on a silicon on insulator platform with 250-nm Si on a 3 ìm buried oxide layer. Fabrication was performed using electron beam lithography followed by reactive ion etching and plasma enhanced chemical vapour deposition of the SiO 2 overcladding. The average width of the right and left sinusoidally modulated waveguides which make up the dispersive gratings are 500 nm and 400 nm, respectively. The amplitude of modulation is 50 nm and 30 nm for the right and left waveguides, respectively. The peak-to-peak separation distance between waveguides is 80 nm. The mean period of modulation is Λ 0 =316 nm for the transmission band to be centred at around 1.545 μm. The total linear chirping period is ΔΛ=3 nm, and is identical in each waveguide, leading to a period, , where , z is the longitudinal coordinate and L is the grating length. The sidewall modulation amplitude of each waveguide is apodized using a filter of the form, f ( z )=(1+0.7 cos(2 π·z/L )−0.3 cos(4 π · z / L ))/1.4. Measurement and calculation of pulse FWHM and peak output power The output pulse FWHM was obtained from the autocorrelation FWHM assuming a Gaussian deconvolution factor of 1.41. Because of the limited autocorrelator scanning range of 15 ps, we were unable to accurately measure the autocorrelation FWHM of the pulse at the lowest peak input power (~100 mW). Therefore, we estimated a minimum pulse FWHM of 7 ps using the measured pulse bandwidth (0.5 nm) corresponding to a time bandwidth product of 0.44. The output peak power from the pulse compressor was calculated using, , where P ave is the average power measured, ν is the laser repetition rate of 76 MHz, P ( t ) is the normalized pulse intensity assuming a Gaussian profile with pulse FWHM obtained from the measured autocorrelation, and f is the estimated fraction of energy carried in the main lobe. The average output power from the nonlinear pulse compressor was measured using a power metre. To calculate the ratio of output to input peak power, the peak output power is normalized to the measured propagation and coupling losses. How to cite this article: Tan, D.T.H. et al . Monolithic nonlinear pulse compressor on a silicon chip. Nat. Commun. 1:116 doi: 10.1038/ncomms1113 (2010).